Strongly enhanced flux pinning in one-step deposition of BaFe2(As0.66P0.33)2superconductor films with uniformly dispersed BaZrO3nanoparticles The high upper critical field and low anisotropy of the iron-based superconductor BaFe 2 As 2 make it promising for its use in the construction of superconducting magnets. However, its critical current density in high magnetic fields needs to be improved. Here we demonstrate a simple, one-step and industrially scalable means of achieving just this. We show that introducing controlled amounts of uniformly dispersed BaZrO 3 nanoparticles into carrier-doped BaFe 2 As 2 significantly improves its superconducting performance without degrading its structural or superconducting properties. Our BaFe 2 (As 0.66 P 0.33 ) 2 films also exhibit an increase in both the irreversibility line and critical current density at all magnetic-field orientations. These films exhibit nearly isotropic critical current densities in excess of 1.5 MA cm −2 at 15 K and 1 T—seven times higher than previously reported for BaFe 2 As 2 films. The vortex-pinning force in these films reaches ~59 GN m −3 at 5 K and 3–9 T, substantially higher than that of the conventional Nb 3 Sn wire. In the search for new classes of superconductors that might replace NbTi and NbSn 3 , the new iron-based superconductors, in particular carrier-doped BaFe 2 As 2 (Ba122), have attracted much attention, as they exhibit high upper critical field [1] and low anisotropy [2] . The powder-in-tube technology has been progressing well for K-doped Ba122 (Ba122:K) and Co-doped Ba122 (Ba122:Co) wires [3] , [4] . However, their critical current density ( J c ) values in a magnetic field are still low, thus indicating the need for flux pinning improvement. As an alternative technology, some groups have indicated the potential of biaxially textured thin-film processing for Ba122:Co-coated conductors [5] , [6] . Although these Ba122:Co films show relatively high J c at self-field ( J c s.f. ) of over 1 MA cm −2 at 4.2 K (because of low misorientation angles at grain boundaries), J c decays rather rapidly when a magnetic field is applied. The decrease in J c in a magnetic field depends on the ability of pinning flux lines, which is determined by the defects that have to be tailored into the material without degrading the current pathway. Indeed, flux pinning has been also one of the most important topics in high-temperature superconductors, such as REBa 2 Cu 3 O y (RE=rare-earth elements; RE123) for electric-power applications [7] , [8] , [9] , [10] , [11] , [12] , [13] . Following the well-known technique of heavy ion irradiation [14] , recently, amorphous tracks induced by heavy-ion irradiation in Ba122:K single crystals [15] were shown to enhance J c at high fields. This irradiation resulted in a matching field as high as 21 T, with no critical temperature ( T c ) degradation. Although heavy-ion irradiation is not practical for long-length wire and tape applications, this work shows that Ba122:K can tolerate a very high density of defects without significant crystalline degradation. However, films of Ba122:K are unlikely to be made in situ because of the high vapour pressure of K. On the other hand, irradiation with protons and heavy ions in Ba122:Co showed clear negative effects in terms of T c degradation [16] , [17] , [18] . Several Ba122:Co films showed strong c axis pinning because of naturally introduced nanopillars, or defects, which can increase J c around the c axis direction [19] , [20] , [21] , without a big improvement around the ab -plane orientation. The naturally occurring defects are difficult to control, indicating the need of a controllable, tunable and practical way to increase vortex pinning in Ba122 films in an isotropic way. Following the outstanding achievements for cuprates [7] , [8] , [9] , [10] , [11] , [12] , [13] , the addition of second phases is a potentially useful technique here. However, in iron-based pnictides, FeAs is known to have a great tendency to segregate at grain boundaries, thus becoming a blocking phase [22] . In order to contribute to the current transport, the second phase needs to be chemically stable and crystallographically compatible, and its size should be sufficiently small to avoid blocking of the current path. Here we report a new one-step strategy that leads to an oxide second phase, resulting in a strong vortex pinning landscape for P-doped Ba122 superconductor films. This is developed on the basis of the easily scalable pulsed laser deposition (PLD) technique. The artificial vortex pinning centres originate from a very dense array of BaZrO 3 (BZO) nanoparticles randomly dispersed within BaFe 2 (As 0.66 P 0.33 ) 2 (Ba122:P) films with virtually no degradation of T c . We chose Ba122:P because it has a T c of ~30 K [23] , higher than that of Ba122:Co [5] , [6] , and is chemically more stable than Ba122:K [24] . Angle-dependent J c ( H , T ) measurements demonstrate that the new strategy is highly effective in preventing vortex motion at high fields, at both 5 and 15 K and for all magnetic-field orientations. A remarkably high pinning force, well over the values for low-temperature superconductors at 4.2 K, is also achieved at both 5 and 15 K. Uniformly dispersed BaZrO 3 in BaFe 2 (As 0.66 P 0.33 ) 2 films Epitaxial BZO-doped Ba122:P (Ba122:P+BZO) thin films (thickness ~80 nm) were grown from 1 mol.% and 3 mol.% BZO-doped PLD targets, and their microstructure was studied by different techniques (see Methods). Spectral maps of Fe, As, Zr, Ba and P for a Ba122:P+3 mol.%BZO film are shown in Fig. 1a–e , respectively, with Fig. 1f showing a cross-sectional transmission electron microscopy (TEM) image. From these images, the presence of uniformly dispersed nanoparticles can be observed. These particles are rich in Zr and poor in Fe, As and P. Ba appears to be homogenously distributed through the film’s thickness; this and the Zr-rich zones suggest the presence of a Ba-Zr-containing phase. The spectral maps yield an average nanoparticle size of ~8 nm with an average spacing L ~24 nm, leading to a density n ~6.8 × 10 22 m −3 . XRD patterns in Fig. 2a indicate that the doped film shows a peak consistent with the BaZrO 3 (110) peak, also consistent with the spectral image of Zr and Ba. As the (200) peak of BZO almost overlaps the (200) peak of the MgO single crystal substrate, it was not possible to conclude about epitaxial film orientation. Figure 2b shows a cross-sectional high-resolution TEM image of the Ba122:P+3 mol.%BZO film, where the electron beam is along <010> of the Ba122:P matrix. 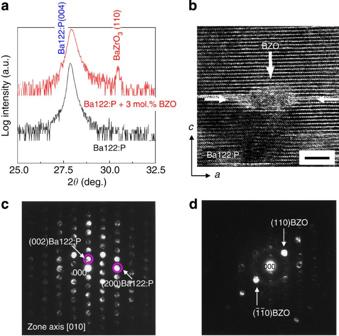Figure 2: Microstructural characterization of a Ba122:P+BZO film. (a) Out-of-planeθ-2θ, X-ray diffraction patterns of Ba122:P and Ba122:P+3mol.%BZO films. The BaZrO3phase is identified in only film with BZO. (b) Cross-sectional high-resolution TEM image of the Ba122:P+3mol.%BZO film, in which a BZO nanoparticle with the height and diameter of ~ 5 and ~ 10 nm, respectively (vertical arrow) can be easily discerned within the matrix. The horizontal arrows point to stacking faults observed around the nanoparticle. The horizontal bar scale indicates 5 nm for (b). (c) Diffraction pattern of the Ba122:P matrix showing that the matrix is coherent with the MgO substrate. (d) Nano-beam diffraction pattern of the BZO nanoparticle showing that it is not coherent with the Ba122:P matrix. A BZO nanoparticle can be clearly discerned within the matrix, its size being ~5 and ~10 nm parallel and perpendicular to the c axis, respectively (vertical arrow). Moreover, a slight strain is observed in the ab- plane around the nanoparticle, similar to what is observed in some RE123 films with nanoparticles [25] . In turn, the periodicity of Ba122 planes around the BZO nanoparticle is only perturbed by the creation of stacking faults (horizontal arrows). Further identification of these nanoparticles is achieved using nano-beam diffraction ( Fig. 2c,d ). Diffraction patterns of the Ba122:P matrix shown in Fig. 2c indicate that the Ba122:P matrix is epitaxially oriented on the MgO substrate. On the other hand, for the BZO nanoparticle (see Fig. 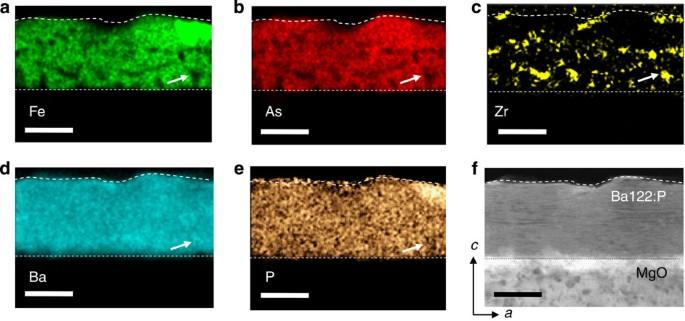2d ), we confirm a diffraction spot of the [110] for BZO—that is, the <110> of BZO is tilted from the <010> of the Ba122:P matrix; the BZO nanoparticles are not epitaxially oriented along the Ba122:P matrix. Figure 1: Cross-sectional elemental maps of a Ba122:P+BZO film. Elemental maps of the Ba122:P+3 mol. %BZO film for Fe, As, Zr, Ba and P, (a–e), respectively. (f) Cross-sectional low-magnification TEM image. The arrows in (a–e) indicate dispersed Ba-Zr-containing nanoparticles. Each horizontal bar indicates 50 nm scale. Figure 1: Cross-sectional elemental maps of a Ba122:P+BZO film. Elemental maps of the Ba122:P+3 mol. %BZO film for Fe, As, Zr, Ba and P, ( a – e ), respectively. ( f ) Cross-sectional low-magnification TEM image. The arrows in ( a – e ) indicate dispersed Ba-Zr-containing nanoparticles. Each horizontal bar indicates 50 nm scale. Full size image Figure 2: Microstructural characterization of a Ba122:P+BZO film. ( a ) Out-of-plane θ -2 θ , X-ray diffraction patterns of Ba122:P and Ba122:P+3mol.%BZO films. The BaZrO 3 phase is identified in only film with BZO. ( b ) Cross-sectional high-resolution TEM image of the Ba122:P+3mol.%BZO film, in which a BZO nanoparticle with the height and diameter of ~ 5 and ~ 10 nm, respectively (vertical arrow) can be easily discerned within the matrix. The horizontal arrows point to stacking faults observed around the nanoparticle. The horizontal bar scale indicates 5 nm for ( b ). ( c ) Diffraction pattern of the Ba122:P matrix showing that the matrix is coherent with the MgO substrate. ( d ) Nano-beam diffraction pattern of the BZO nanoparticle showing that it is not coherent with the Ba122:P matrix. Full size image Table 1 shows a summary of crystallographic and superconducting properties for the Ba122:P and several Ba122:P films with BZO. The superconducting transition temperature ( T c,zero ) of the films was determined by means of electrical transport measurements and is ~26 K for the Ba122:P film, whereas a slightly lower T c (~1 K lower) is observed for the films where BZO was added. This decrease is independent of the BZO percentage added and does not affect the crystalline quality of the matrix as seen in Table 1 . Even though the Ba122:P+BZO films have slightly lower T c s, the J c s.f. s are significantly higher. The J c s.f. of Ba122:P+3 mol.%BZO films at 5 and 15 K are >5 and 3 MA cm −2 , respectively. These J c s.f. values are almost as high as those of Ba122:K single crystals irradiated with a dose of B φ =21 T 15 and higher than those of Ba122:Co films [17] . Table 1 Structural and superconducting properties. 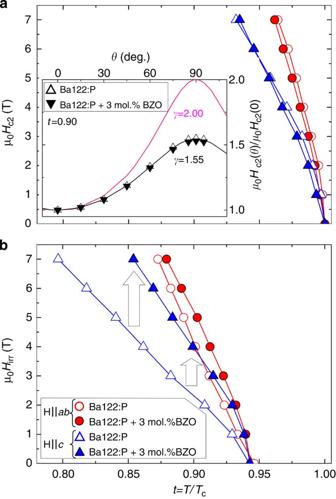Figure 3: Upper critical fieldHc2(T) and irreversibility fieldHirr(T). (a) Normalized temperature (t=T/Tc) dependence ofHc2for Ba122:P and Ba122:P+3mol.%BZO films atH||candH||ab. Inset: angular dependence ofHc2att=0.90 for Ba122:P and Ba122:P+3mol.%BZO films follow a curve consistent withγ~1.55. (b) Normalized temperature dependence ofHirratH||candH||ab. Full size table Upper critical field and improved irreversibility field Figure 3a shows the normalized temperature ( t = T / T c ) dependence of the upper critical field, H c2 for H || c and H || ab for the Ba122:P and Ba122:P+3 mol.%BZO films. H c2 is remarkably similar for both films in spite of their very different pinning landscapes, as is also observed in cuprate superconductors where the coherence length is very small. We extracted the superconducting mass anisotropy ( γ Η ) using anisotropic scaling [26] and found that the films with and without BZO can be described well with γ H ~1.50, which is slightly smaller than γ H for Ba122:Co and Sr122:Co films at the same temperatures [21] , [27] , [28] . These values are in good agreement with the γ ~1.55 value extracted from the angular dependence of H c2 ( t =0.90) for the Ba122:P film and the Ba122:P+3 mol.%BZO film (see inset of Fig. 3a ). Figure 3: Upper critical field H c2 ( T ) and irreversibility field H irr ( T ). ( a ) Normalized temperature ( t = T / T c ) dependence of H c2 for Ba122:P and Ba122:P+3mol.%BZO films at H || c and H || ab . Inset: angular dependence of H c2 at t =0.90 for Ba122:P and Ba122:P+3mol.%BZO films follow a curve consistent with γ ~1.55. ( b ) Normalized temperature dependence of H irr at H || c and H || ab . Full size image The Ba122 films show a small but sizable vortex liquid region between H c2 and the irreversibility field H irr , where J c =0. Reducing the vortex liquid region is of great interest, as it expands the ‘useful’ vortex phase diagram. In Fig. 3b , we show the H irr – t diagram at H || c and H || ab . Although H irr increases slightly after the BZO addition for H || ab , H irr shows a striking increase for H || c . The increase is such that H irr (Ba122:P+3 mol.%BZO) at low fields parallel to the c axis is as high as for H || ab and higher than H irr (Ba122:P) for any orientation. The improvement is maximized around μ 0 H ~3 T, where the intervortex distance is a f ~28 nm, which is close to the average distance between BZO nanoparticles ( L ~24 nm) observed in TEM. This suggests that the maximum reduction in the vortex liquid region occurs when the intervortex spacing corresponds to the distance between nanoparticles. The drastic shrinkage in the vortex liquid phase is very promising and is much more beneficial than that observed in cuprates. Dramatically high J c with nearly isotropic angular dependence In Fig. 4a , we show the field dependence of J c ( H || c ) at 5 K for the reference and BZO-added Ba122:P films. We highlight two major results here; one, that the J c s.f. increases monotonically with the amount of BZO additive (also see Table 1 ) and that the field decay of J c is greatly reduced within the measured field range, indicating a massive improvement in vortex pinning. Further analysis allows us to find the key indicators pointing to the area and reasons for improvement. For Ba122:P films, we observe at low fields that J c is nearly constant up to a characteristic crossover field H * (90% of J c ( H )/ J c s.f. ), followed by a power-law regime ( J c ∝ H − α ) at intermediate fields. Finally, at yet higher fields a more rapid decay of J c is observed as H approaches H irr . For the Ba122:P film, we find α ~0.40 at both 5 and 15 K, which is close to but slightly smaller than the values observed in typical RE123 films with weak point-like defects [29] . 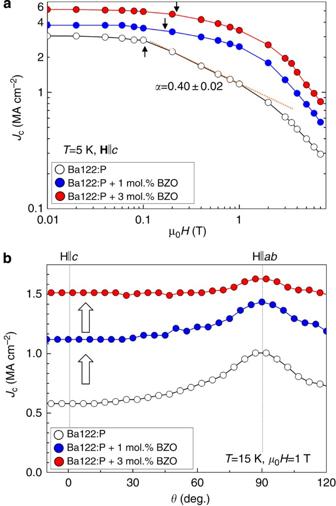Figure 4: Critical current density as a function of magnetic field and angle. (a)Jc(H||c) at 5 K for Ba122:P+1mol.%BZO and Ba122:P+3mol.%BZO films compared with the Ba122:P film. The arrows indicate the positions of the crossover fieldH*. (b) Angular dependence ofJcat 15 K, 1 T for Ba122:P and Ba122:P films with BZO. Figure 4: Critical current density as a function of magnetic field and angle. ( a ) J c ( H || c ) at 5 K for Ba122:P+1mol.%BZO and Ba122:P+3mol.%BZO films compared with the Ba122:P film. The arrows indicate the positions of the crossover field H *. ( b ) Angular dependence of J c at 15 K, 1 T for Ba122:P and Ba122:P films with BZO. Full size image We now turn our attention to the Ba122:P+BZO films. Besides the increase in J c s.f. , H * also increases with BZO content (see arrows in Fig. 4a ). This increase in H * for films with BZO nanoparticles is consistent with the typical effect of nanoparticles [30] , [31] , as the low-field regime is determined to be the single vortex pinning regime. At intermediate fields, we find that both films with BZO show a slower decay of J c ( H ), indicative of the importance of BZO nanoparticles to enhance J c ( H ) in a magnetic field. This improvement in J c ( H ) is manifested such that J c ( H ) does not follow a power-law dependence as in the Ba122:P standard film. This type of non-power-law dependence is similar to that observed in RE123 films, with strong pinning coming from uniformly dispersed nanoparticles [11] , [12] , [32] , [33] . Further insight into the effects of the BZO addition to the pinning landscape of the Ba122:P films can be obtained from the angular-dependent J c . Figure 4b shows J c ( θ ) curves measured for the three films at 1 T, 15 K. Upon addition of BZO, J c increases for all orientations with respect to the J c of the Ba122:P film. Similar to J c s.f. , the improvement is cumulative with increasing BZO content; the increase in J c for the Ba122:P+3 mol.%BZO film is 2.6 times higher than that of the Ba122:P film. It is worth noting that for our Ba122:P+3 mol.%BZO film, we achieve a J c,min of 1.5 MA cm −2 at 1 T, 15 K, which is over 28 times and 7 times higher than that of Ba122:Co films with c axis columnar defects [19] and Ba122:Co films with superlattice structures [34] , respectively, in very similar field and temperature conditions. Moreover, the J c value of the Ba122:P+3 mol.%BZO film is almost the same as that of proton-irradiated Ba122:Co films at 1 T, despite the former being over 10 K higher in temperature [17] . The remarkable in-field performance of Ba122:P films with BZO is highlighted in Fig. 5 , where the pinning force, F p = J c ( H ) × μ 0 H is compared with that of several superconductor materials. At 15 K, F p is over three times higher for the Ba122:P+3 mol.%BZO film than for the Ba122:P film and higher than NbTi [35] at 4.2 K at all magnetic fields; we also find that F p is clearly higher for μ 0 H >0.5 T when compared with MgB 2 data at 15 K [36] . At T =5 K, the F p of the Ba122:P+3 mol.%BZO film reaches ~59 GN m −3 for μ 0 H >3 T up to the highest field we measured (9 T)—a 50% increase over Nb 3 Sn at 4.2 K [37] . This F p value is comparable to that of the RE123-coated conductor with BZO nanoparticles at 65 K 38 . Please note that because the pinning landscape is produced by nanoparticles (and not c axis-oriented nanorods), F p measured along the c axis is just the minimum value for a given field. 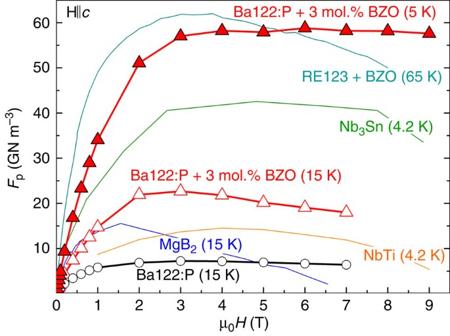Figure 5: Pinning forceFpfor various superconducting materials. TheFp-μ0Hcurves of Ba122:P+3mol.%BZO film at 5 and 15 K and the Ba122 film at 15 K. For comparison, the data for NbTi35at 4.2 K, MgB2(H||ab)36at 15 K, Nb3Sn37at 4.2 K and RE123+BZO-coated conductor38at 65 K are included. Figure 5: Pinning force F p for various superconducting materials. The F p -μ 0 H curves of Ba122:P+3mol.%BZO film at 5 and 15 K and the Ba122 film at 15 K. For comparison, the data for NbTi [35] at 4.2 K, MgB 2 (H|| ab ) [36] at 15 K, Nb 3 Sn [37] at 4.2 K and RE123+BZO-coated conductor [38] at 65 K are included. Full size image Simple analysis tool of vortex pinning by nanoparticles One important aspect of engineering a pinning landscape is the ability of tuning it for maximizing the performance at a particular desired field. One way to characterize the effect of a given pinning improvement route is to calculate the J c enhancement ratio. This of course needs to be performed starting with a state of the art reference sample, the ‘standard’. In Fig. 6a , we present the field dependence of the ratio J c,BZO / J c,standard for Ba122:P films at t=T/T c =0.20 and t =0.60. As for the validity/universality of this approach, we also plot the ratio for RE123 films with a similar density of BZO nanoparticles at the same fields and very similar t . We observe that the J c ratios for the Ba122:P films at both temperatures are very similar, with a maximum around μ 0 H (Δ J c,max )~3.5 T ( H (Δ J c,max ) is the field value at the maximum Δ J c = J c,BZO / J c,standard ). For the case of RE123, the J c ratio exhibits a significant enhancement at μ 0 H (Δ J c,max ) ~3.0 T at high temperatures only, and no clear improvement is found at low temperatures. The similarity of the ratio increase between RE123 at t =0.70 and Ba122:P is remarkable, both in the peak position and amplitude. This result also points out that the BZO inclusions seem to be more effective in Ba122 than in RE123 and in a wider temperature range. 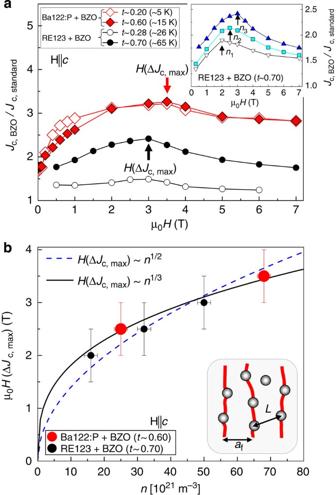Figure 6: Field and nanoparticle-density behaviour of theJcratio. (a) TheJcratio (ΔJc=Jc,BZO/Jc,standard) atH||cfor Ba122:P films att~0.2 andt~0.6. For comparison, the data for RE123 films att~0.28 andt~0.70 are included. Inset:Jc,BZO/Jc,standardatt~0.70 andH||cfor RE123 with different BZO nanoparticle densities (n1=1.6 × 1022,n2=3.1 × 1022andn3=5.0 × 1022m−3). (b) Solid symbols,H(ΔJc,max) atH||cfor Ba122:P films att~0.60; open symbols,H(ΔJc,max) atH||cfor RE123 films att~0.70. Inset: Schematic of a possible configuration of each vortex line is pinned by an array of nanoparticles. Vertical error bars were determined by the magnetic field-measuring intervals; horizontal ones represent the dispersion of the density value obtained from different TEM images. Figure 6: Field and nanoparticle-density behaviour of the J c ratio. ( a ) The J c ratio (Δ J c = J c , BZO / J c , standard ) at H || c for Ba122:P films at t ~0.2 and t ~0.6. For comparison, the data for RE123 films at t ~0.28 and t ~0.70 are included. Inset: J c,BZO / J c,standard at t ~0.70 and H || c for RE123 with different BZO nanoparticle densities ( n 1 =1.6 × 10 22 , n 2 =3.1 × 10 22 and n 3 =5.0 × 10 22 m −3 ). ( b ) Solid symbols, H (Δ J c,max ) at H || c for Ba122:P films at t ~0.60; open symbols, H (Δ J c,max ) at H || c for RE123 films at t ~0.70. Inset: Schematic of a possible configuration of each vortex line is pinned by an array of nanoparticles. Vertical error bars were determined by the magnetic field-measuring intervals; horizontal ones represent the dispersion of the density value obtained from different TEM images. Full size image This difference in effectiveness stems from the nanoparticle size relative to the vortex core size at different temperatures. The BZO nanoparticles in the Ba122:P films are d ~8 nm in diameter, which is a good size to pin a vortex core given its size at either 5 K (2 ξ ab ~5 nm, d /2 ξ ab =1.6) or 15 K (2 ξ ab ~8 nm, d /2 ξ ab =1.0). The BZO nanoparticles in RE123 films are bigger with diameter d ~25 nm. Thus, d /2 ξ ab =3.1 (2 ξ ab ~8.1 nm) at 65 K, which is still effective but not as much as in Ba122:P films. At low temperatures, the size of these particles in RE123 films is much larger than the vortex cores with d /2 ξ ab =5.0 (2 ξ ab (26 K)~5.0 nm), resulting in no significant pinning enhancement even at densities as high as n =5.0 × 10 22 m −3 . These results lead us to deduce that the maximum nanoparticle size for effective pinning needs to be no larger than d /2 ξ ab ( T ) ≅ 3. As mentioned above, H (Δ J c,max ) is temperature-independent for Ba122:P with BZO and has a value very close to that found for RE123 at high t , for a film with a similar BZO nanoparticle density. Indeed, the intervortex distances for μ 0 H (Δ J c,max )=3.5 and 3.0 T (see Fig. 6a ) are 26 and 28 nm, respectively, which are very close to the interparticle spacing determined using TEM of ~24 and ~27 nm, respectively. Furthermore, this correlation is reinforced by the results shown in the inset of Fig. 6a , where a clear increase in H (Δ J c,max ) is observed with increasing density of BZO nanoparticles for RE123 films. These results indicate that H (Δ J c,max ) increases monotonically with increasing particle density. This is further reflected in Fig. 6b , where H (Δ J c,max ) is plotted against n for Ba122:P ( t ~0.60) and RE123 ( t ~0.70) films. A clear universal dependence of H (Δ J c,max ) on n is observed for both types of films. This dependence can be fitted with a power law, such that H (Δ J c,max )~ n 1/3~1/2 . The latter dependence is consistent with the observation that a f ~ L . This is shown schematically in the inset of Fig. 6b , in which the vortex line separation is the same as the distance between nanoparticles. This indicates that the maximum improvement in J c produced by the BZO nanoparticle additions occurs when the elastic energy (that is, vortex repulsive interactions) of the vortices is minimized to accommodate to the strong pinning exerted by the nanoparticles. This phenomenological model is valid in the density range of technological interest and leads to μ 0 H (Δ J c,max )=0 for no added particles. Koshelev et al. [39] studied theoretically the effect of an array of nanoparticles on the vortex line pinning and found that the critical current is determined by the length of the trapped segment, leading to L ∝ n . In this model, the critical force grows roughly as n 1/2 . From the experimental results and the theoretical analysis above, we find a simple but effective rule for optimizing the performance of a material at a given magnetic field for both iron-pnictides and cuprates with nanoparticles. Namely, process the material to yield nanoparticles with average size smaller than ~3 × (2 ξ ( T )) and with densities such that the nanoparticle spacing matches the intervortex distance at the given magnetic field H (Δ J c,max ). For application to magnets, an isotropic field angular dependence of J c is as important as its value. A significant increase in J c around the c axis direction was reported for the Ba122:Co films with naturally introduced nanopillars (or defects) [19] , [20] , [21] . Although Ba122:Co films with superlattice structures were recently shown to have an improved J c not only in the c axis but also in the ab -plane directions, the angular dependence of J c is still anisotopic [34] . We achieved a notably high J c,min with nearly isotropic angular dependence (the ratio J c,max / J c,min =1.1) by simply adding BaZrO 3 nanoparticles. The present achievement offers a method for developing novel superconducting tapes, and possibly cables, with a simple one-step deposition and industrially scalable production process that can be used to make high-field magnets for operation in the temperature range up to 15 K. At the same time, our simple analysis tool allows the application of this method to any superconductor for better tuning and engineering of the critical current improvements. The drastic reduction in the extend of vortex liquid phase region and large isotropic critical current obtained indicate a fruitful route for improving other iron-pnictide materials. Rethinking the role of the superconducting matrix and its ability of withstanding large amounts of material defects and inclusions is also critical to increasing vortex pinning without blocking superconducting currents. Thus, an important effort should be concentrated in this area both in iron- and copper-based superconductors. PLD target preparation for BaFe 2 (As 0.66 P 0.33 ) 2 films Polycrystalline PLD targets with the nominal compositions of BaFe 2 (As 0.66 P 0.33 ) 2 , BaFe 2 (As 0.66 P 0.33 ) 2 +1 mol.% BaZrO 3 and BaFe 2 (As 0.66 P 0.33 ) 2 +3 mol.% BaZrO 3 were sintered following standard procedures. As starting materials, Ba metal (99.99%, chunk), Fe metal (99.9%, no. 300 mesh pass), As powder (99.9999%,~3 μm grain) and P powder (99.999%, no. 600 mesh pass) were used. Processing was carried out in an argon-filled glove box. Ba metal was cut into small pieces to promote reaction. Ba and As at a ratio of 1:1 were put into an alumina tube. It was sealed in an evacuated quartz tube and heat-treated at 500 °C for 10 h and 650 °C for 20 h. A similar procedure was carried out for FeAs 0.17 P 0.33 in nominal composition. The reacted materials were pulverized using an agate mortar and mixed together in a ratio of BaAs:FeAs 0.17 P 0.33 =1:2. The powder mixture was press-formed into a pellet, reacted at 650 °C for 10 h and 900 °C for 24 h in an evacuated quartz tube. Then, 1 and 3 mol% of BaZrO 3 powder (Toshima Manufacturing Co. Ltd) were added to the above BaFe 2 (As 0.67 P 0.33 ) 2 powder, reacted at 1,000 °C for 24 h. BaFe 2 (As 0.66 P 0.33 ) 2 films with BaZrO 3 nanoparticles Epitaxial films (~80 nm in thickness) were deposited on MgO (100) single crystal substrates by ablating the polycrystalline PLD targets using the second harmonic (wavelength: 532 nm) of a pulsed Nd:YAG laser at a repetition rate of 10 Hz in vacuum of 10 −4 Pa at a substrate temperature of 800 °C. Film thickness was measured from cross-sectional TEM images at several points and ranged from 72 to 80 nm. Transport properties in magnetic fields Films were patterned using photolithography and ion milling into bridges of ~50 μm width. The crystalline quality was examined using XRD. The temperature dependence of the resistivity ( ρ ) was measured by a four-probe method in the temperature range of 10–300 K using a Quantum Design PPMS with a superconducting magnet generating a field H of up to 9 T. In the PPMS, a rotational stage was used to rotate the samples with respect to H . The H c2 and H irr were determined using 0.90 ρ N and 0.01 ρ N criteria, respectively, where ρ N is the normal-state resistivity. The critical current was determined using a 1 μV cm −1 criterion. Microstructure and chemical composition analysis The microstructures and elemental concentration mappings of the films were analysed by TEM and energy-dispersive X-ray spectroscopy, respectively. How to cite this article: Miura M. et al. Strongly enhanced flux pinning in one-step deposition of BaFe 2 (As 0.66 P 0.33 ) 2 superconductor films with uniformly dispersed BaZrO 3 nanoparticles. Nat. Commun. 4:2499 doi: 10.1038/ncomms3499 (2013).